The mTORC1 effectors S6K1 and 4E-BP play different roles in CNS axon regeneration Using mouse optic nerve (ON) crush as a CNS injury model, we and others have found that activation of the mammalian target of rapamycin complex 1 (mTORC1) in mature retinal ganglion cells by deletion of the negative regulators, phosphatase and tensin homologue (PTEN), and tuberous sclerosis 1 promotes ON regeneration. mTORC1 activation inhibits eukaryotic translation initiation factor 4E-binding protein (4E-BP) and activates ribosomal protein S6 kinase 1 (S6K1), both of which stimulate translation. We reasoned that mTORC1’s regeneration-promoting effects might be separable from its deleterious effects by differential manipulation of its downstream effectors. Here we show that S6K1 activation, but not 4E-BP inhibition, is sufficient to promote axon regeneration. However, inhibition of 4E-BP is required for PTEN deletion-induced axon regeneration. Both activation and inhibition of S6K1 decrease the effect of PTEN deletion on axon regeneration, implicating a dual role of S6K1 in regulating axon growth. Permanent loss of vital functions after central nervous system (CNS) injury occurs in part because axons in the adult mammalian CNS do not regenerate [1] , [2] , [3] . Growth failure is due to the diminished intrinsic regenerative capacity of mature neurons [4] and to the inhibitory environment of the adult CNS [5] . We and others have found that activation of the mammalian target of rapamycin complex 1 (mTORC1) in adult retinal ganglion cells (RGCs) by deletion of the negative regulators, phosphatase and tensin homologue (PTEN), and tuberous sclerosis 1 (TSC1) promotes optic nerve (ON) regeneration after crush injury [6] . Similar findings have been reported for mammalian cortical motor [7] and peripheral sensory neurons [8] , [9] , drosophila sensory neurons [10] and Caenorhabditis elegans motor neurons [11] , suggesting that mTORC1 is a neuron intrinsic regulator of axon regeneration. mTOR is a serine/threonine protein kinase that interacts with other proteins to form a functional complex, mTORC1, which acts as a key downstream signal of the phosphatidylinositol 3-kinase (PI3K)-AKT pathway to regulate cell growth, proliferation, metabolism, motility and survival [12] , [13] . The TSC1/TSC2 heterodimer is a major upstream inhibitor of mTORC1 that can be phosphorylated and inhibited by AKT to activate mTORC1. Phosphatase and tensin homologue (PTEN) is a lipid phosphatase that converts phosphatidylinositol (3,4,5)-triphosphate to phosphatidylinositol 4,5-bisphosphate and thus inhibits the activation of downstream effectors of PI3K. Deletion of PTEN or TSC therefore results in constitutive aberrant activation of mTORC1, thereby playing a central role in tumorigenesis, metabolic diseases and neurological disorders [13] , [14] . Because of the increasing evidence that the PTEN/mTORC1 pathway can regulate axon regeneration [4] , [6] , [7] , [8] , [9] , [10] , [11] , [15] , [16] , [17] , [18] , mTORC1 and its downstream effectors are logical therapeutic targets for enhancing axon regeneration and functional recovery after neural injury. The two best-characterized downstream signalling molecules of mTORC1 are ribosomal protein S6 kinase (S6K) and eukaryotic translation initiation factor 4E (eIF4E)-binding protein (4E-BP) [19] . Phosphorylation of 4E-BP by mTORC1 releases its binding from eIF4E, enabling incorporation of eIF4E into eIF4F complex to initiate cap-dependent translation. S6K also promotes protein and lipid synthesis [20] , [21] and its full activation requires phosphorylation of both T389 by mTORC1 and T229 by PI3K-phosphoinositide-dependent kinase-1 (ref. 22 ). Although 4E-BP inhibition and S6K activation are both downstream of mTORC1 activation, and both promote protein synthesis, previous studies suggested that S6K and 4E-BP differentially control cell growth and proliferation: S6K controls cell size but not cell cycle progression [23] , whereas 4E-BP controls cell proliferation but not cell size [24] . In the present study, we have used the ON crush model because its axons project in a single direction, which insures that any nerve fibres observed distal to a complete crush injury have regenerated and do not represent spared axons that underwent collateral sprouting or efferent axons from the brain to the retina. Our findings confirm S6K1’s effect on neuronal cell size and identify its regeneration-promoting and regeneration-inhibiting roles after CNS axon injury. In contrast to S6K1 activation, inhibition of 4E-BP is not sufficient for axon regeneration, but it is necessary for PTEN deletion-induced axon regeneration. Our studies reveal the complicated cross-regulating mechanisms by which PTEN/mTORC1 signalling controls axon regeneration and point out clear future directions for differentiating the regeneration-promoting effects of mTORC1 from its deleterious effects. S6K1 activation promotes RGC survival and ON regeneration The two members of the mammalian S6K family (S6K1 and S6K2) are ubiquitously expressed in all tissues and share 84% identity in their kinase domains [22] . However, their functions are not redundant because S6K1 KO mice are 20% smaller than WT mice, and S6K2 KO mice are slightly larger [22] . The strikingly reduced size of pancreatic β-cells and myoblast cells in S6K1 KO mice is part of the evidence suggesting a role of S6K1, but not S6K2, in determining cell size [23] , [25] , [26] . Consistent with this notion, S6K1/2 double KO (DKO) mice are similar in size to S6K1 single KO mice [27] , and a constitutively active (CA) mutant of S6K1 (T389E-D3E) rescues the size of S6K1/2 DKO cells even in the presence of mTOR inhibitor [23] , [28] . Therefore, to understand the role of S6K in axon regeneration, we focused on S6K1 rather than S6K2. We used the S6K1-CA mutant (T389E-D3EE) and the dominant-negative (DN) mutant (T229A) of S6K1 to manipulate S6K1 activity in mouse RGCs [29] . We first confirmed that S6K1 mutants produce the expected changes in S6K1 activity in transfected HEK293 cells in vitro ( Supplementary Fig. 1a ): The 40S ribosome protein S6 (S6) is a direct substrate of S6K and the phosphorylated form of S6 (pS6) is a reliable marker for mTORC1 and S6K activation. Overexpression of WT S6K1 or S6K1-CA mutant significantly increased pS6 levels, whereas S6K1-DN decreased them. Next, we used adeno-associated virus (AAV2) to express S6K1 mutants in vivo, since we and others have demonstrated a specific tropism of AAV2 for RGCs after intravitreal injection [6] , [30] , [31] , [32] . We generated AAV2 vectors that contained CAG promoter-driven hemagglutinin (HA)-tagged S6K1-CA and S6K1-DN. These viruses showed >90% infection efficiency, and their effects on pS6 levels in RGCs were similar to those in vitro, based on triple labelling of HA (S6K1 tag), Tuj1 (antibody for RGC marker, β-III tubulin) and pS6 (indicator of S6K1 activity) in whole-mount retina ( Supplementary Fig. 1b ). We then performed ON crush in WT mice 2 weeks after intravitreal injection of AAV-S6K1 mutants. S6K1-CA increased and S6K1-DN decreased RGC cell size significantly, demonstrated by co-injection of AAV-GFP ( Supplementary Fig. 2 ), consistent with its function in cell size control. We also evaluated RGC survival based on Tuj1 staining in retinal whole mounts. At 2 weeks post crush, S6K1-CA increased peripheral RGC survival to 36%, compared with only 23% in WT control mice ( Fig. 1a,b ). Downregulation of S6K1 activity by S6K1-DN did not further reduce RGC survival (21%; Fig. 1a,b ). RGC axons that regenerated through the lesion site were labelled anterogradely by intravitreal injection of the tracer Alexa 488-conjugated cholera toxin-β (CTB), and imaged in ON longitudinal sections. Similar to their effects on RGC survival, expression of S6K1-CA, but not S6K1-DN, resulted in significant axon regeneration in WT mice ( Fig. 1c,d ). Thus, the mTORC1 downstream effector, S6K1, promoted both peripheral RGC survival and ON regeneration. 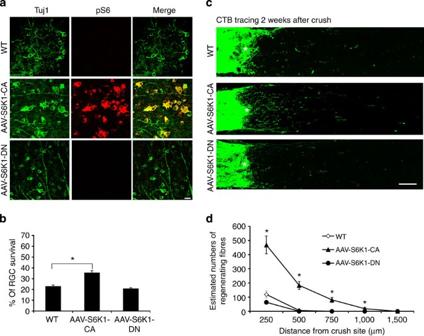Figure 1: S6K1 activation promotes axon regeneration and RGC survival. (a) Confocal images of flat-mounted retinas showing surviving Tuj1-positive RGCs and pS6 immunostaining, 2 weeks after ON crush. Scale bar, 20 μm. (b) Quantification of surviving RGCs, represented as percentage of Tuj1-positive RGCs in the injured eye, compared with the intact contralateral eye. *P≪0.001. Data are presented as means±s.e.m.,n=8–12. (c) Confocal images of ON longitudinal sections showing regenerating fibres labelled with CTB 2 weeks after ON crush. *Crush site. Scale bar, 100 μm. (d) Quantification of regenerating fibres at different distances distal to the lesion site. *P≪0.001. Data are presented as means±s.e.m.,n=8–12. Figure 1: S6K1 activation promotes axon regeneration and RGC survival. ( a ) Confocal images of flat-mounted retinas showing surviving Tuj1-positive RGCs and pS6 immunostaining, 2 weeks after ON crush. Scale bar, 20 μm. ( b ) Quantification of surviving RGCs, represented as percentage of Tuj1-positive RGCs in the injured eye, compared with the intact contralateral eye. * P ≪ 0.001. Data are presented as means±s.e.m., n =8–12. ( c ) Confocal images of ON longitudinal sections showing regenerating fibres labelled with CTB 2 weeks after ON crush. *Crush site. Scale bar, 100 μm. ( d ) Quantification of regenerating fibres at different distances distal to the lesion site. * P ≪ 0.001. Data are presented as means±s.e.m., n =8–12. Full size image 4E-BP inhibition is not sufficient for ON regeneration We next tested the influence of another downstream effector of mTORC1, 4E-BP, on RGC survival and axon regeneration. There are three 4E-BP genes in mouse: 4E-BP2 is the predominant isoform in the brain, with only low levels of 4E-BP1 and no detectable 4E-BP3 (ref. 19 ). Since phosphorylation by mTORC1 reduces the activity of 4E-BP, we performed ON crush in 4E-BP 1 and 2 DKO (4E-BP1/2 DKO) mice [33] . 4E-BP KO had no effect on pS6 level ( Fig. 2a ), and thus did not affect endogenous S6K activity. Similar to S6K1 activation, 4E-BP1/2 DKO mice showed a statistically significant, although small increase (28%) in peripheral RGC survival ( Fig. 2a,b ). However, we failed to observe any enhancement of ON regeneration in 4E-BP1/2 DKO mice ( Fig. 2c,d ), suggesting that, despite its small increase of cell survival, 4E-BP inhibition is not sufficient for axon regrowth. To determine whether S6K1 and 4E-BP act synergistically, we performed ON crush after intravitreal injection of AAV-S6K1-CA into 4E-BP1/2 DKO mice. There was no significant increase of RGC survival compared with 4E-BP KO alone ( Fig. 2b ) or of ON regeneration compared with S6K1 activation alone ( Figs 1d and 2d ). Taken together, our results suggest that 4E-BP inactivation promotes survival of injured RGC, but is not sufficient to allow CNS axon regeneration. 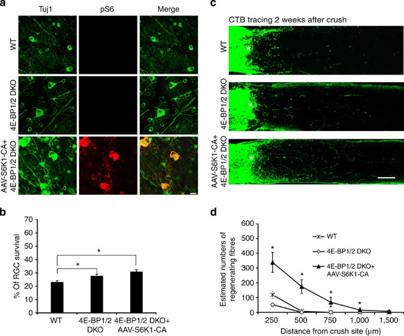Figure 2: 4E-BP1/2 deletion increases RGC survival but has no effect on axon regeneration. (a) Confocal images of flat-mounted retinas showing surviving Tuj1-positive RGCs and pS6 immunostaining, 2 weeks after ON crush. Scale bar, 20 μm. (b) Quantification of surviving RGCs, represented as percentage of Tuj1-positive RGCs in the injured eye, compared with the intact contralateral eye. *P≪0.05. Data are presented as means±s.e.m.,n=8–12. (c) Confocal images of ON longitudinal sections showing regenerating fibres labelled with CTB 2 weeks after ON crush. *Crush site. Scale bar, 100 μm. (d) Quantification of regenerating fibres at different distances distal to the lesion site. *P≪0.05. Data are presented as means±s.e.m.,n=8–12. Figure 2: 4E-BP1/2 deletion increases RGC survival but has no effect on axon regeneration. ( a ) Confocal images of flat-mounted retinas showing surviving Tuj1-positive RGCs and pS6 immunostaining, 2 weeks after ON crush. Scale bar, 20 μm. ( b ) Quantification of surviving RGCs, represented as percentage of Tuj1-positive RGCs in the injured eye, compared with the intact contralateral eye. * P ≪ 0.05. Data are presented as means±s.e.m., n =8–12. ( c ) Confocal images of ON longitudinal sections showing regenerating fibres labelled with CTB 2 weeks after ON crush. *Crush site. Scale bar, 100 μm. ( d ) Quantification of regenerating fibres at different distances distal to the lesion site. * P ≪ 0.05. Data are presented as means±s.e.m., n =8–12. Full size image The additive effect of S6K1 and SOCS3 on ON regeneration Axons regenerate more robustly in PTEN/SOCS3 (suppressor of cytokine signalling 3) DKO mice than in either single KO alone [15] , indicating an additive effect of these two pathways. We therefore tested whether S6K1 activation (downstream of PTEN/mTORC1) in SOCS3 KO mice results in more axon regeneration than in the SOCS3 KO alone. First, we confirmed that transgene expression and Cre-mediated conditional gene deletion in RGCs are highly efficient by injecting a 1:1 mixture of AAV-Cre and AAV-HA-transgene into a reporter mouse line. This mouse line contains a LoxP-stop codon-LoxP-GFP and expresses GFP upon Cre expression. More than 80% of Tuj1+RGCs expressed both GFP (Cre expression reporter) and HA (transgene tag; Supplementary Fig. 3a ). Next we confirmed that S6K1-CA injection significantly increased pS6 levels in SOCS3 KO mice ( Supplementary Fig. 3b ). We then performed ON crush in the same cohorts of SOCS3-floxed mice injected with AAV-Cre (dilute 1:1 with PBS) alone or with AAV-S6K1-CA+AAV-Cre. Although there was no significant difference in survival of RGC ( Fig. 3a,b ), S6K1 activation together with SOCS3 deletion induced more robust axon regeneration than SOCS3 KO alone ( Fig. 3c,d ) or S6K1-CA alone (compared with Fig. 1c,d ). This result suggests that S6K1 may contribute to the additive effect observed in PTEN/SOCS3 DKO mice [15] . 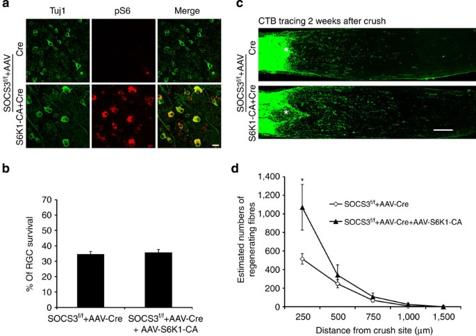Figure 3: S6K1 activation and SOCS3 deletion act additively to promote axon regeneration. (a) Confocal images of flat-mounted retinas showing surviving Tuj1-positive RGCs and pS6 immunostaining, 2 weeks after ON crush in SOCS3f/fmice injected with either AAV-Cre or AAV-Cre +AAV-S6K1-CA. Scale bar, 20 μm. (b) Quantification of surviving RGCs, represented as percentage of TUJ1-positive RGCs in the injured eye, compared with the intact contralateral eye, 2 weeks after ON crush. Data are presented as means±s.e.m. (c) Confocal images of ON longitudinal sections showing regenerating fibres labelled with CTB 2 weeks after ON crush. *Crush site. Scale bar, 100 μm. (d) Quantification of regenerating fibres at different distances distal to the lesion site. *P≪0.05. Data are presented as means±s.e.m.,n=8–12. Figure 3: S6K1 activation and SOCS3 deletion act additively to promote axon regeneration. ( a ) Confocal images of flat-mounted retinas showing surviving Tuj1-positive RGCs and pS6 immunostaining, 2 weeks after ON crush in SOCS3 f/f mice injected with either AAV-Cre or AAV-Cre +AAV-S6K1-CA. Scale bar, 20 μm. ( b ) Quantification of surviving RGCs, represented as percentage of TUJ1-positive RGCs in the injured eye, compared with the intact contralateral eye, 2 weeks after ON crush. Data are presented as means±s.e.m. ( c ) Confocal images of ON longitudinal sections showing regenerating fibres labelled with CTB 2 weeks after ON crush. *Crush site. Scale bar, 100 μm. ( d ) Quantification of regenerating fibres at different distances distal to the lesion site. * P ≪ 0.05. Data are presented as means±s.e.m., n =8–12. Full size image The dual role of S6K1 in PTEN KO-induced ON regeneration To directly investigate the role of S6K1 in PTEN deletion-induced axon regeneration, we blocked S6K1 activity by intravitreal injection of AAV-S6K1-DN+AAV-Cre in PTEN-floxed mice. Compared with the very low activity of mTORC1/S6K (low pS6 level) in adult WT mice, and the moderate increase in pS6 level after PTEN deletion, S6K1-DN significantly reduced pS6 levels in PTEN KO mice ( Supplementary Fig. 4 ). Consistent with the downregulation of S6K1 activity, S6K1-DN significantly decreased RGC survival ( Supplementary Fig. 5 ) and axon regeneration in PTEN KO mice ( Fig. 4a,b ), indicating that the PTEN KO effect depends at least partially on S6K1 activity. We also co-injected AAV-S6K1-CA+AAV-Cre in PTEN-floxed mice and detected an increased pS6 level ( Supplementary Fig. 4 ). We were surprised to find, however, that, rather than increasing RGC survival or axon regeneration, S6K1 over-activation in PTEN KO mice did not increase RGC survival ( Supplementary Fig. 5 ) and significantly decreased axon regeneration ( Fig. 4a,b ). These findings suggest that S6K1 activation also plays an inhibitory role in the regeneration induced by PTEN KO. S6K1 participates in a negative feedback loop of insulin receptor/PI3K signalling, that is, by phosphorylating insulin receptor substrate 1, it reduces activities of PI3K and downregulates phosphorylation of AKT [34] , [35] . Consistent with its action in this system, levels of phosphorylated AKT were lower in PTEN KO mice after S6K1-CA injection ( Fig. 4c ). Taken together, these results revealed a dual role of S6K1 in CNS axon regeneration: its activation is sufficient to promote axon regeneration, whereas it inhibits PTEN deletion-induced axon regeneration through feedback inhibition of the PI3K pathway. 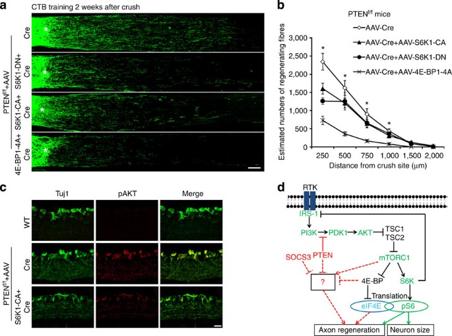Figure 4: Both S6K1 and 4E-BP are involved in PTEN deletion-induced axon regeneration. (a) Confocal images of ON longitudinal sections showing regenerating fibres labelled with CTB, 2 weeks after ON crush. *Crush site. Scale bar, 100 μm. (b) Quantification of regenerating fibres at different distances distal to the lesion site. *P≪0.05. Data are presented as means±s.e.m.,n=8–12. (c) Confocal images of retina cross-sections immunostained with Tuj1 and phosphorylated AKT (pAkt) antibodies, 2 weeks after AAV injection. Scale bar, 20 μm. (d) Schematic summary of the PTEN/mTORC1 signalling pathways in CNS axon regeneration. The dashed lines represent the possible cross talk among these pathways. The question mark represents unknown effectors downstream of these pathways that contribute to CNS axon regeneration. Figure 4: Both S6K1 and 4E-BP are involved in PTEN deletion-induced axon regeneration. ( a ) Confocal images of ON longitudinal sections showing regenerating fibres labelled with CTB, 2 weeks after ON crush. *Crush site. Scale bar, 100 μm. ( b ) Quantification of regenerating fibres at different distances distal to the lesion site. * P ≪ 0.05. Data are presented as means±s.e.m., n =8–12. ( c ) Confocal images of retina cross-sections immunostained with Tuj1 and phosphorylated AKT (pAkt) antibodies, 2 weeks after AAV injection. Scale bar, 20 μm. ( d ) Schematic summary of the PTEN/mTORC1 signalling pathways in CNS axon regeneration. The dashed lines represent the possible cross talk among these pathways. The question mark represents unknown effectors downstream of these pathways that contribute to CNS axon regeneration. Full size image 4E-BP inhibition is required for PTEN KO-induced ON regeneration Although 4E-BP KO does not allow axon regeneration, we evaluated whether phosphorylation/inhibition of 4E-BP is required for axon regeneration in PTEN KO mice. We expressed HA-tagged 4E-BP1-4A mutant using AAV in RGCs ( Supplementary Fig. 6 ). This mutant cannot be phosphorylated by mTORC1 and therefore binds to eIF4E to inhibit translation constitutively [36] . In the same cohorts of PTEN-floxed mice injected with AAV-Cre (diluted 1:1 with PBS) or AAV-Cre+AAV-4E-BP1-4A, ON regeneration was significantly reduced in the eyes with 4E-BP1-4A expression ( Fig. 4a,b ), indicating the 4E-BP phosphorylation/inhibition by mTORC1 is necessary for PTEN KO-induced axon regeneration. The S6K and 4E-BP pathways are both downstream of mTORC1 and both are involved in mRNA translation and protein synthesis, but in non-neuronal cells, S6K and 4E-BP exert different effects on cell growth and proliferation. The results of the present study showed that S6K1 and 4E-BP also have distinct effects on CNS axon regeneration. S6K1 activation, but not 4E-BP inhibition, was sufficient for axon regeneration. Thus, these two translational control mechanisms downstream of mTORC1 contribute to CNS axon regeneration in different ways, presumably through different translational targets. The amount of axon regeneration induced by S6K1 was much smaller than that of PTEN deletion, suggesting that S6K1 activation mediates only part of the effect of PTEN KO. The additive effect of S6K1 and SOCS3 further supports the notion that S6K1 is involved in the axon regeneration induced by PTEN deletion. Identification of the complete set of S6K1 substrates will be required to better understand how S6K1 regulates axon regeneration. Interestingly, S6K1 phosphorylates and inhibits GSK3 in an AKT-independent manner [37] . Since inhibition of GSK3 has been suggested to promote axon regeneration [38] , [39] , which is also AKT independent [40] , GSK3 is an obvious candidate effector of S6K1 for axon regeneration. S6K1 also can phosphorylate and inhibit fragile X mental retardation protein (FMRP), an RNA-binding protein that prevents mRNA translation [41] . However, we did not detect significant ON regeneration in FMR1 (FMRP gene) KO mice (unpublished data). Another substrate of S6K1 is BAD, a pro-apoptotic BH3-only molecule of the Bcl-2 family, through which S6K1 may promote cell survival [42] . By phosphorylation of insulin receptor substrate 1, S6K1 participates in a negative feedback loop of insulin/insulin receptor/PI3K signalling that reduces activities of PI3K and its downstream effectors ( Fig. 4d ) [13] , [22] , [34] , [35] . TSC deletion results in high S6K1 activity and low AKT activity owing to S6K1’s feedback inhibition of PI3K (refs 34 , 37 ). Thus, an explanation for the unexpected inhibitory effect of S6K1 activation on axon regeneration may be that the increased S6K1 activity after S6K1-CA expression reduces PI3K-AKT signalling in PTEN KO mice and therefore inhibits PI3K-dependent and S6K1-independent axon regeneration. The decreased phosphorylated AKT levels observed in PTEN KO RGCs after S6K1-CA expression support this idea. This mechanism, higher mTORC1/S6K1 activity inhibiting PI3K-AKT signalling, might also account for the smaller amount of axon regeneration in TSC1 KO mice, as S6K1 activity is much higher in TSC1 KO mice compared with that in PTEN KO mice [6] . As we were preparing this manuscript, a new publication reported that S6K inhibits axon regeneration in C. elegans [43] . Our results demonstrate that the inhibitory role of S6K1 on axon regeneration is conserved in mammals, although we also reveal that mammalian S6K1 can exert a markedly opposite stimulatory action on CNS axon regeneration. Thus, the axon regeneration that we saw in AAV-S6K1-CA injected WT mice ( Fig. 1 ) may result from the combination of S6K1’s growth-promoting and growth-inhibiting effects, which are exerted through different substrates. 4E-BP inhibition alone did not allow axon regeneration and together with S6K1 activation only partially reproduced the axon regeneration induced by PTEN KO /mTORC1 activation, suggesting that other substrates of mTORC1 (refs 44 , 45 ) or other effectors of PTEN may also contribute to axon regrowth ( Fig. 4d ). These effectors remain to be identified. The significant reduction in axon regeneration in PTEN KO mice after overexpression of CA 4E-BP (4E-BP1-4A), however, indicates the necessity of 4E-BP phosphorylation/inhibition downstream of mTORC1 for axon regeneration, either through its specific translational targets or through other unknown mechanisms. In summary, our study provides evidence that differential translational control of mTORC1 is a critical determinant of the neuron’s intrinsic growth ability. S6K1-dependent signalling, PTEN/PI3K-dependent but S6K1-independent effectors, uncharacterized substrates of mTORC1 (refs 44 , 45 ) and 4E-BP-dependent targets may act cohesively to guide axon regeneration. The identification of these effectors will warrant future investigation. Mice PTEN flox/flox , SOCS3 flox/flox and C57BL/6 WT mice were purchased from Jackson Laboratories (Bar Harbor, Maine). 4E-BP1/2 DKO mice were obtained from Dr Nahum Sonenberg’s laboratory [33] . All mice were of C57BL/6 background male and 5- to 7–week old at the time of surgery. All breeding and experimental procedures were performed in compliance with animal protocols approved by the Institutional Animal Care and Use Committee (IACUC) at Temple University School of Medicine. For all surgical and treatment comparisons, controls and treatment groups were prepared together in single cohorts, and the experiment repeated at least twice. AAV production The constructs of the CA mutant (T389E-D3EE) and DN mutant (T229A) of p70S6K1 were obtained from Dr George Thomas’s laboratory [29] , and the 4E-BP1-4A mutant was obtained from Addgene (no. 382400). We subcloned into an AAV backbone with CAG promoter. An HA or Myc tag was added at the N terminus of the transgene as a marker for its expression. To generate and package recombinant AAV particles, AAV plasmids containing the transgenes were co-transfected with pAAV-RC (Stratagene) and the pHelper plasmid (Stratagene) into HEK293T cells. Seventy-two hours after transfection, the cells were lysed to release the viral particles, which were then precipitated by 40% polyethylene glycol and purified by caesium chloride density gradient centrifugation. The fractions with refractive index from 1.370 to 1.374 were taken out for dialysis in MWCO 7000 Slide-A –LYZER cassette (Pierce) overnight at 4 °C. The AAV titres used for this study were in the range of 1.5–2.5 × 10 12 genome copies per millilitre determined by real-time PCR. Intravitreal injection and ON crush For each intravitreal injection, the micropipette was inserted in the peripheral retina just behind the ora serrata; it was deliberately angled to penetrate into the vitreous chamber without damaging the lens. Approximately 2 μl of the vitreous was removed before injection of 2 μl AAV into the vitreous chamber. ON crush was performed as described previously [6] , [31] . In brief, 2 weeks following AAV injection, the left ON was exposed intraorbitally and crushed with jeweler’s forceps (Dumont no. 5; Fine Science Tools) for 5 s ~0.5 mm behind the eyeball. Care was taken not to damage the underlying ophthalmic artery. Eye ointment containing atropine sulphate was applied to protect the cornea after surgery. RGC axon anterograde tracing Two microlitres of CTB conjugated with fluorescence Alexa 488 (2 μg μl −1 , Invitrogen) was injected into the vitreous chamber 2 days before killing the animals to label the regenerating axons in the ON. Animals were killed by CO 2 and fixed by perfusion with 4% paraformaldehyde in cold PBS. Eyes with the nerve segment still attached were dissected out and post fixed in the same fixative for another 2 h at room temperature. Tissues were cryoprotected through increasing concentrations of sucrose (15–30%) and optimal cutting temperature compound (Tissue Tek), then snap-frozen on dry ice. Serial longitudinal cross-sections (8 μm) were cut and stored at –80 °C until processed. Immunohistochemistry of whole-mount retina Retinas were dissected out from 4% paraformaldehyde fixed eyeballs and washed extensively in PBS before blocking in staining buffer (10% normal goat serum and 2% Triton X-100 in PBS) for half an hour. All antibodies were diluted in the same staining buffer. Antibodies used were as follows: mouse neuronal class β-III tubulin (clone Tuj1, 1:500 dilution; Covance), rat HA (clone 3F10, 1:100 dilution, Roche) and pS6 rabbit antibody (1:400, Cell Signaling). Floating retinas were incubated with primary antibodies overnight at 4 °C and washed three times for 30 min each with PBS. Secondary antibodies (Cy2-, Cy3- or Cy5-conjugated) were then applied (1:200–400; Jackson ImmunoResearch) and incubated for 1 h at room temperature. Retinas were again washed three times for 30 min each with PBS before a cover slip was attached with Fluoromount-G (SouthernBiotech). Immunohistochemistry of retina cross-sections PFA (4%)-fixed eyes were dehydrated with increasing concentrations of sucrose solution (15–30%) overnight and embedded in optimal cutting temperature on dry ice. Serial cross-sections (12 μm) were cut with a Leica cryostat and collected on Superfrost Plus Slides. The retina sections were blocked in the staining buffer (10% normal goat serum and 0.1% Triton X-100 in PBS) for 30 min followed by primary antibody staining. The following antibodies were used: mouse neuronal class β-III tubulin (clone Tuj1, 1:500 dilution; Covance), phospho-AKT-Ser473 (193H12, 1:200 dilution; Cell Signaling). The sections were incubated with primary antibodies overnight at 4 °C and washed three times for 15 min each with PBS. Secondary antibodies (Cy2, Cy3 conjugated) were then applied (1:200–400; Jackson ImmunoResearch) and incubated for 1 h at room temperature. Sections were again washed three times for 15 min each with PBS before a cover slip was attached with Fluoromount-G (SouthernBiotech). Counting surviving RGCs and regenerated axons For RGC counting, whole-mount retinas were immunostained with the Tuj1 antibody and 6–9 fields were randomly sampled from peripheral regions of each retina. The percentage of RGC survival was calculated as the ratio of surviving RGC numbers in injured eyes compared with contralateral uninjured eyes. For axon counting, the number of CTB-labelled axon was obtained by counting the fibres crossing perpendicular lines drawn on ON sections distal to the crush site at intervals of 250 μm for the first 1,000 μm, and then at intervals of 500 μm until no fibres were visible. The width of the nerve (R) was measured at the point (d) at which the counts were taken and were used together with the thickness of the section ( t =8 μm) to calculate the number of axons per μm 2 area of the nerve. The formula used for the calculation was ∑ad= πr 2 × (axon number)/( R × t ). The total number of axons per section was then averaged over three sections per animal. All CTB signals in the range of intensity that was set from lowest to maximum after background subtraction were counted as individual fibres by Nikon NIS Element R4 software. Counts of surviving cells and regenerated axons were performed by a single observer who was blinded with regard to the surgical manipulations and treatments. Statistical analyses Data are presented as means±s.e.m with 8–12 mice per experimental group. We used one-way analysis of variance with Bonferroni’s post hoc test for multiple comparisons. How to cite this article: Yang, L. et al. The mTORC1 Effectors S6K1 and 4E-BP Play Different Roles in CNS Axon Regeneration. Nat. Commun. 5:5416 doi: 10.1038/ncomms6416 (2014).